Osmotic-pressure-controlled concentration of colloidal particles in thin-shelled capsules Colloidal crystals are promising structures for photonic applications requiring dynamic control over optical properties. However, for ease of processing and reconfigurability, the crystals should be encapsulated to form ‘ink’ capsules rather than confined in a thin film. Here we demonstrate a class of encapsulated colloidal photonic structures whose optical properties can be controlled through osmotic pressure. The ordering and separation of the particles within the microfluidically created capsules can be tuned by changing the colloidal concentration through osmotic pressure-induced control of the size of the individual capsules, modulating photonic stop band. The rubber capsules exhibit a reversible change in the diffracted colour, depending on osmotic pressure, a property we call osmochromaticity. The high encapsulation efficiency and capsule uniformity of this microfluidic approach, combined with the highly reconfigurable shapes and the broad control over photonic properties, make this class of structures particularly suitable for photonic applications such as electronic inks and reflective displays. Colloidal crystals exhibit unique optical properties; the size of each colloidal particle is comparable to the wavelength of light, and their periodic arrangement in a colloidal crystal leads to selective diffraction of light, thereby producing structural colours [1] , [2] , [3] , [4] . As the optical properties are determined by the interparticle separation [5] , the photonic properties can be dynamically modulated. Such dynamic control is especially useful for reflective colour displays, which have been fabricated by embedding colloidal particles in a polymer matrix whose swelling is controlled by an external electric field [6] , [7] . Dynamic control of diffraction has also be exploited to create colorimetric biosensors that change their structural colour upon specific binding of a biomolecule [8] , [9] , [10] , [11] , [12] , [13] . In all of these cases, the modulation of the photonic properties is controlled by changing the interparticle spacing, which requires fluid to flow out from the crystal; this transport is limited by diffusion, and thus rapid response requires small dimensions. Typically, this is achieved by preparing thin films of colloidal crystals. More rapid modulation of photonic properties can be achieved by crystalline colloidal arrays, which are generated by interparticle repulsion in a liquid phase; electric or magnetic field can lead to the compression or relaxation of the crystals, thereby providing dynamic control of structural colours [14] , [15] . However, these formats limit the ease with which these photonic structures can be processed, thereby restricting their potential uses. One way to overcome this limitation is to confine colloidal crystals in emulsion drops. To make such encapsulated crystals, the droplets must first be formed at a low volume fraction of particles and then the solvent should be removed from the interior typically through evaporation [16] , [17] , [18] , until the particles form a closely packed spherical crystal. However, it is difficult to control the evaporation rate while maintaining droplet stability; moreover, the photonic structure is not reconfigurable and the dynamic control is lost. Thus, there remains a need for a new type of encapsulated colloidal crystal structure that enables easy processibility, reconfigurability, easily modulated photonic properties and dynamic control of structural colours. In this article, we use capillary microfluidics to controllably produce photonic capsules containing a suspension of colloidal crystals that can be dynamically reconfigured. We first encapsulate colloidal particles in double-emulsion drops with ultra-thin shells. The thin membrane facilitates transport of water into or out of the droplet when it is subjected to an osmotic pressure difference. This allows the concentration of particles within the drops to be controlled precisely yet varied rapidly through external driving. By controlling the concentration in this way, we can create dramatic changes in the appearance of the capsules, including pronounced iridescence or sparkling colours. The photonic liquid capsules can be further stabilized by polymerizing monomers in the membrane, leading to a shell with tunable rigidity. In the flexible photonic capsules, the volume and hence structural colour can be controlled by the osmotic pressure, a property we call osmochromaticity; moreover, the internal structures can be adjusted to produce crystalline or amorphous structures depending on the rate of change of their volume, providing additional flexibility in controlling the photonic properties. Finally, the high flexibility of the capsules and their spherical shape make them highly reconfigurable and easily processed while allowing them to be packed with low void fraction. When the capsules are deformed, the colloidal particles can rearrange by aligning their crystal planes along the inner wall of the membrane. In addition, the high mobility of the colloidal crystals confined in the capsules allows rapid modulation of the structural colours through external fields, making the capsules useful for various photonic devices [14] , [15] . Microfluidic encapsulation and concentration We prepare double-emulsion drops with ultra-thin shells through emulsification of a core-sheath flow in a capillary microfluidic device. Two immiscible fluids are injected through a single capillary channel, and the fluid with higher affinity to the wall flows along the capillary, while the other fluid flows through the centre of the channel without contacting the wall. This forms a core-sheath flow that can be emulsified in the continuous phase, producing double-emulsion drops with ultra-thin shells [19] . For example, using 10 wt.% aqueous solution of polyvinyl alcohol (PVA) as both the innermost and the continuous phases, and ethoxylated trimethylolpropane triacrylate (ETPTA) as the middle oil phase, we generate water-in-oil-in-water liquid capsules with a 750-nm-thick liquid membrane. The strong lubrication resistance in the membrane stabilizes the core-shell structure by significantly retarding migration of the inner drops; this dramatically reduces contact between the inner and outer interfaces, therefore increasing the lifetime of the capsules [20] . Transport of water across the membrane can be precisely controlled by the osmolarity of the continuous phase. Under hypertonic conditions, where the osmolarity of the continuous phase is higher than that of the inner phase, the drop shrinks isotropically. During this shrinkage, the thickness of the oil liquid membrane increases while the osmotic pressure difference decreases, leading to a decay of the water flux. Ultimately, the drops reach isotonic conditions when the osmotic pressure difference becomes negligible, as schematically illustrated in Fig. 1a . For example, liquid capsules composed of a water core with 100 mOsml −1 and a membrane of ETPTA exhibit isotropic shrinkage in time when they are subjected to an outermost fluid with 460 mOsml −1 , as shown in Fig. 1b and Supplementary Movie 1 . 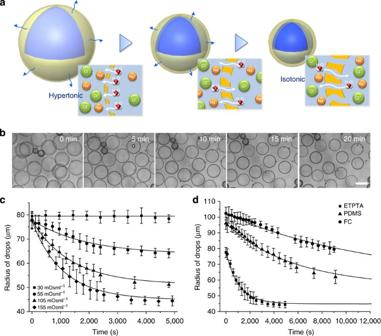Figure 1: Isotropic shrinkage of liquid capsules. (a) Schematic illustration of isotropic shrinkage of a liquid capsule under hypertonic condition; the capsule shrinks until the osmotic pressure difference becomes negligible. (b) A series of optical microscope images showing isotropic shrinkage of liquid capsules consisting of 10 wt.% aqueous core of PVA with 100 mOsml−1and ETPTA membrane, where the capsules are dispersed in aqueous solution with 460 mOsml−1. Scale bar, 100 μm. (c) Time dependence of radius of liquid capsules with 750-nm-thick ETPTA membrane dispersed in continuous phase with four different osmolarities, where aqueous cores contain 0.5 wt.% PVA and 2.5 wt.% PEG with 30 mOsml−1; fits with equation 2 are shown by solid lines. (d) Time dependence of radius of liquid capsules in continuous phase with 155 mOsml−1, where three different liquid membranes of 750-nm-thick ETPTA, 218-nm-thick PDMS and 104-nm-thick FC oils are used; fits with equation 2 yield diffusivity of water molecule in the oil membrane: 11.0 μm2s−1for ETPTA, 0.723 μm2s−1for PDMS and 0.161 μm2s−1for FC. The error bars inc,dindicate s.d. For a radius R much larger than the shell thickness l , the rate of shrinkage is: Figure 1: Isotropic shrinkage of liquid capsules. ( a ) Schematic illustration of isotropic shrinkage of a liquid capsule under hypertonic condition; the capsule shrinks until the osmotic pressure difference becomes negligible. ( b ) A series of optical microscope images showing isotropic shrinkage of liquid capsules consisting of 10 wt.% aqueous core of PVA with 100 mOsml −1 and ETPTA membrane, where the capsules are dispersed in aqueous solution with 460 mOsml −1 . Scale bar, 100 μm. ( c ) Time dependence of radius of liquid capsules with 750-nm-thick ETPTA membrane dispersed in continuous phase with four different osmolarities, where aqueous cores contain 0.5 wt.% PVA and 2.5 wt.% PEG with 30 mOsml −1 ; fits with equation 2 are shown by solid lines. ( d ) Time dependence of radius of liquid capsules in continuous phase with 155 mOsml −1 , where three different liquid membranes of 750-nm-thick ETPTA, 218-nm-thick PDMS and 104-nm-thick FC oils are used; fits with equation 2 yield diffusivity of water molecule in the oil membrane: 11.0 μm 2 s −1 for ETPTA, 0.723 μm 2 s −1 for PDMS and 0.161 μm 2 s −1 for FC. The error bars in c , d indicate s.d. Full size image where ΔC is the osmolarity difference, P is the permeability of water molecules in the oil membrane and α is the molar volume of water ( α =0.018 lmol −1 ) [21] . Expressing P = D / l ( R ), where D is the diffusivity of water molecules in the oil of the membrane, and using the dependence of ΔC on the osmolarity of the outer fluid, C out , the initial osmolarity in the drop, C 0 , and initial drop radius, R 0 , we have We obtain excellent agreement with equation 2 and data for ETPTA capsules subjected to different values of C out , as shown in Fig. 1c . As expected, increasing osmotic pressure difference leads to more rapid shrinkage, while there is no change in size in the absence of an osmolarity difference. The only fitting parameter is D ; the fits yield values of D that are consistent for different values of C out ; average value of D is 11.3 μm 2 s −1 . The agreement with the model also shows that other effects, such as the Laplace pressure of the capsule, do not significantly affect the transport. This is expected, since even at long times, when the radius of drop approaches R 0 ( C 0 / C out ) 1/3 , the Laplace pressure of the capsules—which is equal to 4γ / R , where γ is the interfacial tension between water and ETPTA (~2.24 mNm −1 ) [22] —is two orders of magnitude less than the osmotic pressure [23] . We can also control the rate of shrinkage by using different oils in the membranes, such as polydimethylsiloxane (PDMS) oil or fluorocarbon (FC) oil. Although capsules made with these membranes exhibit different rates of shrinkage, the transport is well described by equation 2, as shown in Fig. 1d ; from the fits, we estimate values of D of 0.723 μm 2 s −1 for PDMS oil and 0.161 μm 2 s −1 for FC oil. By comparison with weakly polar ETPTA, nonpolar PDMS oil has a value of diffusivity that is 16-fold lower, whereas the very hydrophobic FC oil has a value of diffusivity that is 70-fold lower. This enables us to vary the rate of shrinkage by than two orders of magnitude at the same osmotic pressure difference. Concentration and crystallization of colloids in capsules We use the osmotic pressure to control the concentration of colloidal particles confined within the liquid capsules and thereby modulate the photonic properties. As an internal phase, we use an aqueous suspension of polystyrene (PS) particles with diameter, d , of 175 nm and initial volume fraction, φ 0 , of 0.093 containing 2 wt.% PVA. Poly( N -isopropylacrylamide) (pNIPAAm) chains are grafted on the surface of the PS to render the particles hydrophilic and prevent them from anchoring to the interfaces of the emulsion [24] . In addition, these grafted chains induce a short-ranged steric repulsion between particles. We use a glass capillary device to generate monodisperse double-emulsion drops with a 400-nm-thick membrane of ETPTA and containing an aqueous core of PS particles, as shown in Fig. 2a,b and Supplementary Movie 2 . The drops are subjected to a higher osmotic pressure and incubated to shrink them and concentrate the particles; subsequently, we polymerize the ETPTA monomers to form a solid membrane. The degree of shrinkage, R / R 0 , and therefore the volume fraction, φ=φ 0 ( R 0 / R ) 3 , is determined by the osmotic pressure and the incubation time; higher pressures and longer times result in smaller capsules with higher φ in the core. 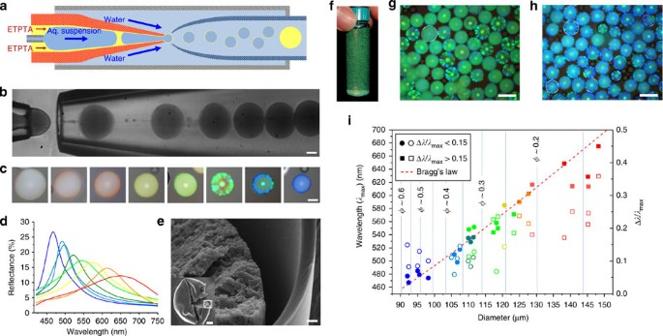Figure 2: Concentration and crystallization of colloids in capsules. (a) Schematic illustration of a capillary microfluidic device for production of double-emulsion drops with ultra-thin membrane. (b) Still shot image showing generation of monodisperse liquid capsules with average diameter of 168 μm containing 175 nm polystyrene particles in their cores at volume fraction,φ0, of 0.093. (c) Optical microscope images of photonic capsules with different diameter and diffraction colour; the capsules are produced by osmotic pressure-induced shrinkage and subsequent photopolymerization of the ETPTA membrane. Scales inb,care set to be same for direct size comparison. Scale bars, 50 μm. (d) Reflectance spectra measured from single photonic capsules with different diameters. (e) Scanning electron microscope (SEM) image of dried and broken photonic capsules; colloidal crystal and cross-section of solid membrane are included in a field of view. Scale bar, 1 μm. Inset shows overall shape of the dried capsules. Scale bar, 20 μm. (f) Aqueous suspension of the photonic capsules displaying green colour. (g,h) Optical microscope images of monodisperse photonic capsules displaying green and blue colours, respectively. Scale bars, 100 μm. (i) Size dependence of peak position,λmax, and normalized full-width at half-maximum, Δλ/λmax, of reflection spectra of the photonic capsules, where solid symbols correspond toλmaxand empty symbols correspond to Δλ/λmax; diameter of capsules determines volume fraction of particles in the core,φ, as shown by vertical lines in the plot. According to value of Δλ/λmax, photonic capsules are classified into two categories: Δλ/λmax<0.15 denoted by circles and Δλ/λmax>0.15 denoted by squares. Dotted line corresponds to Bragg’s diffraction from (111) planes of fcc lattice. Figure 2: Concentration and crystallization of colloids in capsules. ( a ) Schematic illustration of a capillary microfluidic device for production of double-emulsion drops with ultra-thin membrane. ( b ) Still shot image showing generation of monodisperse liquid capsules with average diameter of 168 μm containing 175 nm polystyrene particles in their cores at volume fraction, φ 0 , of 0.093. ( c ) Optical microscope images of photonic capsules with different diameter and diffraction colour; the capsules are produced by osmotic pressure-induced shrinkage and subsequent photopolymerization of the ETPTA membrane. Scales in b , c are set to be same for direct size comparison. Scale bars, 50 μm. ( d ) Reflectance spectra measured from single photonic capsules with different diameters. ( e ) Scanning electron microscope (SEM) image of dried and broken photonic capsules; colloidal crystal and cross-section of solid membrane are included in a field of view. Scale bar, 1 μm. Inset shows overall shape of the dried capsules. Scale bar, 20 μm. ( f ) Aqueous suspension of the photonic capsules displaying green colour. ( g , h ) Optical microscope images of monodisperse photonic capsules displaying green and blue colours, respectively. Scale bars, 100 μm. ( i ) Size dependence of peak position, λ max , and normalized full-width at half-maximum, Δ λ / λ max , of reflection spectra of the photonic capsules, where solid symbols correspond to λ max and empty symbols correspond to Δ λ / λ max ; diameter of capsules determines volume fraction of particles in the core, φ , as shown by vertical lines in the plot. According to value of Δ λ / λ max , photonic capsules are classified into two categories: Δ λ / λ max <0.15 denoted by circles and Δ λ / λ max >0.15 denoted by squares. Dotted line corresponds to Bragg’s diffraction from (111) planes of fcc lattice. Full size image As the particles become concentrated in the core, they display a sequence of colours starting from white and progressing from red to blue, as shown in Fig. 2c and Supplementary Fig. 1 . When the capsule shrinks only small amount, it remains white because of the strong scattering and lack of ordering. As the particle volume fraction progresses to φ ~0.15, the capsule displays a weak reddish colour, suggesting the onset of short-range correlations [25] , [26] . The colour is blue-shifted and becomes more vivid as φ increases with further shrinkage. At φ ~0.25, the capsules display pronounced iridescence or brilliant colours, as shown in the sixth image of Fig. 2c , indicating the onset of long-range order. This evolution in the appearance of the capsule is confirmed by reflectance spectra measured from single capsules, shown in Fig. 2d . The influence of the number density of capsules on the spectra is also included in Supplementary Fig. 2 . Scanning electron micrographs illustrate the ordering at φ ~0.55, as shown in Fig. 2e : the colloidal particles form a face-centred cubic (fcc) lattice whose (111) plane is aligned along the wall of the spherical capsule [16] , [17] . The colour is uniform from droplet to droplet, as shown in Fig. 2f–h and Supplementary Fig. 3 . Some capsules containing crystals exhibit colour patterns or patches on their side surfaces, which are attributed to diffraction from other stacked planes of the fcc lattice due to formation of (111) planes along the spherical surface [27] . The ordering of the particles in the capsules with decreasing size is evidenced by the decrease in the full-width at half-maximum (FWHM) of the reflectance spectra ( Fig. 2i ). For samples with φ >0.25, which are iridescent, the FWHMs of the spectra are narrow, Δλ / λ max <0.15, indicating crystalline order. By contrast, for φ <0.25, the samples do not exhibit any iridescence but nevertheless are strongly coloured. Here the FWHM is broader, indicating strong local ordering of the particles but no long-range crystalline order. The volume fraction where crystallization first occurs, φ c ~0.25, is significantly less than that for hard spheres, φ c ~0.494 (ref. 28 ), indicating a repulsive interaction between particles; we attribute this to steric effect of the grafted pNIPAAm chains. For the crystalline samples, the dependence of λ max on capsule size is nearly linear and agrees with expectations for Bragg diffraction from (111) planes of an fcc lattice ( Fig. 2i ), given by Kim et al . [29] : where n p and n w are the refractive indices of particle and water, respectively. Elastomeric photonic capsules When the ETPTA is polymerized to form a rigid membrane, the capsules no longer respond to osmolarity under hypotonic conditions and instead maintain nearly constant radius. Although the osmotic pressure can drive water molecules into the capsules, the membrane cannot stretch to accommodate them because of its high Young’s modulus, E ~600 MPa [30] . As a result, the colour does not change with osmotic pressure, and the peak positions of the reflection spectra remain unchanged as shown in Fig. 3a,c . Under hypertonic conditions, the solid capsules buckle as water is drawn from the interior through the membrane [31] . This results in 45-nm blue shift of the reflectance peak in the spectra. 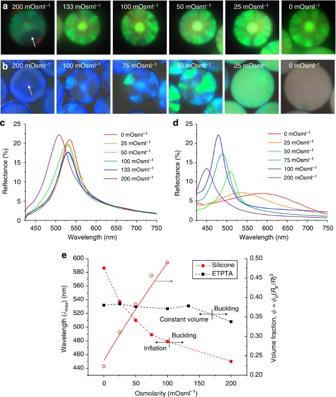Figure 3: Elastomeric photonic capsules. (a,b) Optical microscope images of photonic capsules with a rigid ETPTA and flexible silicone membranes dispersed in aqueous solutions of NaCl with different osmolarities as denoted in the images, respectively. (c,d) Corresponding reflectance spectra of photonic capsules with a rigid and flexible membranes, respectively. (e) Osmolarity dependence of peak position of reflectance spectra,λmax, from photonic capsules consisting of rigid ETPTA membrane (solid squares) and flexible silicone membrane (solid circles). Volume fraction of particles at the core of photonic capsules with silicone membrane,φ, is shown by empty circles in the right axis; a fit with equation 4 yields Young’s modulus of silicone membrane as 6.86 MPa. Figure 3: Elastomeric photonic capsules. ( a , b ) Optical microscope images of photonic capsules with a rigid ETPTA and flexible silicone membranes dispersed in aqueous solutions of NaCl with different osmolarities as denoted in the images, respectively. ( c , d ) Corresponding reflectance spectra of photonic capsules with a rigid and flexible membranes, respectively. ( e ) Osmolarity dependence of peak position of reflectance spectra, λ max , from photonic capsules consisting of rigid ETPTA membrane (solid squares) and flexible silicone membrane (solid circles). Volume fraction of particles at the core of photonic capsules with silicone membrane, φ , is shown by empty circles in the right axis; a fit with equation 4 yields Young’s modulus of silicone membrane as 6.86 MPa. Full size image We create stable, responsive elastomeric capsules by using silicone resin, which polymerizes to form a flexible membrane. Under hypotonic conditions, the capsules behave like balloons: they inflate because of the inward flux of water. Lower osmolarity in the outer fluid leads to larger capsules and lower volume fraction of particles, thereby resulting in a red shift of the structural colour, as shown in Fig. 3b,d and Supplementary Fig. 4 . For low volume fraction, colloidal structures in the core do not possess long-range order and show relatively weak colour and broad reflectance spectra. For hypertonic conditions, the rubber capsules are also buckled because of outward flux of water, resulting in a blue shift of colour in the spectra ( Fig. 3d ). To determine the modulus of the membrane, we consider that in equilibrium, the osmotic pressure should be balanced by the membrane elasticity: where R gas is the gas constant, E is Young’s modulus, A p is the surface area of the capsule at the moment of polymerization and ΔA is the deviation of surface area from A p . To determine ΔC we use to determine ΔA / A p we use and to determine l , we use where C p , R p and l p are the osmolarity of the core, the radius of the capsule and the thickness of the membrane at the moment of polymerization. In addition, we consider the osmolarity dependence of particle volume fraction of the core of the flexible capsules, φ=φ p ( R p / R ) 3 , where φ p is φ at the moment of polymerization, φ p ~0.49. We obtain good agreement in volume fraction, φ , with equation 4 and the data for the rubber capsules, as shown by the solid lines in Fig. 3e . Fitting for the modulus E yields a value of 6.86 MPa, 90-fold smaller than that of ETPTA. Influence of the concentration rate on crystallization We use the flexible photonic capsules to study the influence of the concentration rate on colloidal crystallization. We transfer the rubber capsules from distilled water into aqueous solutions of NaCl with three different concentrations. The capsules all experience an outward flux of water through membrane while maintaining their spherical shape, leading to an increase in particle concentration and a concomitant blue shift of the colour. However, this occurs at different rates depending on the osmotic pressure difference as shown in Fig. 4a–c and Supplementary Movie 3 . The capsule subjected to the lowest osmotic pressure difference exhibits the slowest increase in concentration; in this case, we observe the formation of a central dot and colour patterns at the capsule edge before it ultimately buckles. These colour spots reflect nucleation and growth of colloidal crystals. By contrast, in capsules subjected to higher osmotic pressure differences, crystallization is suppressed. Instead, the colour shifts towards the blue, reflecting the increase in concentration; however, the sample remains disordered, or glass-like, even after buckling. We summarize the time dependence of the particle volume fraction, φ=φ 0 ( R 0 / R ) 3 , in Fig. 4d . 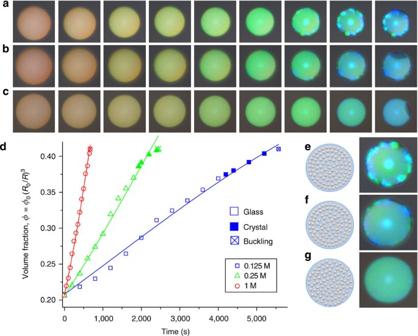Figure 4: Influence of the concentration rate on colloidal crystallization. (a–c) Series of optical microscope images of photonic rubber capsules, which are transferred from distilled water to 0.125, 0.25 and 1 M aqueous solutions of NaCl at the beginning, where images are taken at intervals of 800 s, 400 s and 100 s, respectively. (d) Time dependence of volume fraction of particles in the core of the photonic rubber capsules,φ, where empty symbols correspond to glassy structure, solid symbols correspond to colloidal crystal and cross symbols correspond to buckled capsule; fits on these data with equation 8 yield permeability of water molecules through the membrane,κ, as 4.60 × 10−12, 5.88 × 10−12and 4.89 × 10−12μm2for three cases, which are very closely equal. (e–g) Schematics and optical microscope images of photonic capsules immediately before onset of buckling, which are dispersed in 0.125 M, 0.25 M and 1 M aqueous solutions of NaCl, respectively. The rate of shrinkage of the capsule is described by Darcy’s law with permeability of water through the membrane, κ, where both osmotic pressure and elasticity drive the outward flux during isotropic shrinkage: [31] Figure 4: Influence of the concentration rate on colloidal crystallization. ( a – c ) Series of optical microscope images of photonic rubber capsules, which are transferred from distilled water to 0.125, 0.25 and 1 M aqueous solutions of NaCl at the beginning, where images are taken at intervals of 800 s, 400 s and 100 s, respectively. ( d ) Time dependence of volume fraction of particles in the core of the photonic rubber capsules, φ , where empty symbols correspond to glassy structure, solid symbols correspond to colloidal crystal and cross symbols correspond to buckled capsule; fits on these data with equation 8 yield permeability of water molecules through the membrane, κ , as 4.60 × 10 −12 , 5.88 × 10 −12 and 4.89 × 10 −12 μm 2 for three cases, which are very closely equal. ( e – g ) Schematics and optical microscope images of photonic capsules immediately before onset of buckling, which are dispersed in 0.125 M, 0.25 M and 1 M aqueous solutions of NaCl, respectively. Full size image where μ is viscosity of water. The data are in excellent agreement with the predictions of equation 8, as shown in Fig. 4d . Fits for the membrane permeability, κ , yield consistent values for various values of C out . The response time of the silicone capsules to osmotic pressure differences is on the order of 10 3 s, comparable to that of colorimetric sensors based on polymerized crystalline colloidal arrays [11] . The response can potentially be improved by using elastic membranes with higher permeability. The silicone capsules are highly flexible, enabling deformation of the capsules while maintaining the integrity of the membrane. For example, the capsules can be compressed between two glass slides to make disks, as shown in Supplementary Fig. 5 ; this is different from solid ETPTA capsules, which easily rupture on mechanical compression, as shown in Supplementary Fig. 6 . Upon compression, particles in the silicone capsules rearrange by aligning their crystal planes along the inner surface of the membrane. Thus, the flattened capsules exhibit uniform reflection colour, as shown in Supplementary Fig. 5 . The integrity of membrane of the capsules is maintained until the ratio of diameter to thickness of the disk becomes 7.8. Upon further compression, the membrane ruptures, releasing the colloidal particles into the continuous phase. This high flexibility enables dense packing of the capsules, as shown in Supplementary Fig. 7 ; such low void fractions cannot be achieved by solid capsules and may be useful for display applications where it is necessary to achieve high reflectivity and resolution [32] . In addition, dynamic modulation of the structural colours can potentially be achieved by applying an external electric field, which can compress or relax the liquid-suspended colloidal crystals confined inside the capsules [15] . Photonic capsules with ultra-thin membranes of liquid, rigid solid and elastomer have unique characteristics making them potentially useful for many photonic applications. Liquid capsules provide precise control in concentration of particles, and the liquid membrane can rupture with high sensitivity to external stimuli, potentially leading to a photonic sensor with release functionality. Solid capsules with a rigid shell can retain their photonic properties even when subjected to strong external pressure, making them useful for photonic devices requiring long-term operation. Flexible capsules can be deformed easily, facilitating dense capsule packing with low void fraction and enabling passage through small pores or holes. Such capsules may therefore prove useful for displays and injectable microsensors: dense arrays of capsules can provide high reflectivity and strong structural colours that are potentially tunable with external electric fields, and individual capsules might be used to measure osmotic pressure or detect bioactives. Moreover, the production of such capsules can be scaled up by parallelizing the droplet-making process, as shown in Supplementary Movie 4 . We therefore expect this class of materials, in which the optical properties can be precisely and quantitatively controlled through transport and deformation, to benefit a wide range of applications requiring responsive photonic structures. Materials An aqueous solution of PVA (Mw 13,000–23,000, Sigma-Aldrich) is used as the innermost and the continuous phase of double-emulsion drops, which stabilizes interfaces between water and oil. As middle oil phases, we use one of four solutions: ETPTA (Sigma-Aldrich) containing 0.2 wt.% photoinitiator (2-hydroxy-2-methylpropiophenone, Sigma-Aldrich), polysiloxanes modified with methacrylate (SB4722, ν ( η / ρ )=570 cSt, Evonik) containing 0.2 wt.% photoinitiator, PDMS oil ( ν =20 cSt, Sigma-Aldrich) containing 2 wt.% surfactant (DC749, Dow Corning) and FC oil (3-ethoxy-1,1,1,2,3,4,4,5,5,6,6,6-dodecafluoro-2-trifluoromethyl-hexane, HFE 7500, 3 M) containing 1 wt.% surfactant (Krytox-PEG-Krytox surfactant) [33] ; to produce solid microcapsules, we use ETPTA solution, while we use SB4722 solutions to make rubber capsules. As a collection liquid for double-emulsion drops, we use an aqueous mixture of PVA and NaCl with controlled osmolarity. Polystyrene particles with the diameter of 175 nm are synthesized by emulsion polymerization and treated with PNIPAAm to render them hydrophilic; the PNIPAAm chains are grafted on the surface of particles, stabilizing the suspension of the particle [34] . Zeta potential of the resultant particles is measured as −26 mV (Zetasizer Nano-ZS90, Malvern Instruments). The particles are dispersed in an aqueous solution of PVA; this suspension is used as the innermost phase to produce photonic capsules. Osmolarity of all aqueous solutions is measured using osmometer (Model 3300, Advanced Instruments Inc.) before use. Fabrication of microfluidic device and its operation To make capillary microfluidic devices, two cylindrical glass capillaries of 1 mm in outer diameter (World precision instruments Inc., 1B100-6) are tapered and coaxially assembled in square capillary of 1.05 mm in inner dimension (AIT glass) ( Fig. 2a ); one cylindrical capillary with a 140-μm-diameter orifice is treated with n-octadecyltrimethoxyl silane (Sigma-Aldrich) to render it hydrophobic, whereas the other cylindrical capillary with a 200-μm-diameter orifice is treated with 2-[methoxy(polyethyleneoxy)propyl] trimethoxyl silane (Gelest Inc.) to render it hydrophilic. The separation of these cylindrical capillaries is set to be 150 μm. In addition, small tapered capillary are inserted into the hydrophobic cylindrical capillary through wide opening. To produce double-emulsion drops, the innermost aqueous phase is injected through the small tapered capillary and the middle oil phase is injected through the hydrophobic capillary. The continuous phase is injected through interstices between the hydrophilic and square capillaries as co-current flow to the innermost and middle phases. Flow rates of the innermost, middle and continuous phases are typically set to be 300 μlh −1 , 200 μlh −1 and 3,000 μlh −1 , respectively. In the hydrophobic injection capillary, the innermost phase flows in a form of plug-like drops without contacting the wall, while the middle phase forms a continuous phase. When the plug-like drops arrive at the tip of the injection capillary, such core-sheath flow is emulsified into the continuous phase, producing double-emulsion drops with ultra-thin shell; excess oil between the plug-like drops in the middle phase is not incorporated into the emulsion drops but instead forms large independent oil blobs. Although both double-emulsion drops and oil blobs are generated in this discontinuous production, double-emulsion drops with an ultra-thin shell are easily separated from the mixture by exploiting their density difference. During drop generation, flow rates are controlled by syringe pumps (Harvard Apparatus) and the flow is observed using an inverted microscope equipped with a high-speed camera (Phantom V9.0). Osmosis-induced concentration and polymerization of the membrane The resultant double-emulsion drops are collected in aqueous solutions of PVA and NaCl with controlled osmolarity and incubated at room temperature; the osmolarity, diffusivity of water in the middle oil and incubation time influence on rate of shrinkage. For capsules with a rigid ETPTA membrane in Fig. 3 , liquid capsules containing PS particles and 3 wt.% PVA are incubated in aqueous solution with 170 mOsml −1 for 1 h prior to polymerization. For capsules with a flexible silicone membrane, liquid capsules containing PS particles and 1.7 wt.% PVA are incubated in aqueous solution with 100 mOsml −1 for 24 h, resulting in R p =48 μm and l p =1.42 μm. To analyse time dependence of the drop size, we monitor the drops under optical microscope in a course of incubation, where the chamber is closed to minimize evaporation. To solidify the shell of ETPTA, silicone resin, the monomers are polymerized by ultraviolet exposure for 30 s (Omnicure S1000, 100 W) and the capsules are transferred into distilled water; without the transfer, the capsules are buckled in hypertonic condition. Characterization The photonic microcapsules are observed using an upright microscope (Ni-U, Nikon) and their reflectance spectra are measured using fibre optic spectrometer (USB4000, Ocean Optics). For measurement of the spectra from single capsules, we used a × 50 lens and a field stop on the microscope to exclude contributions from the background fluid; we confirmed that the contribution from the background was negligible by measuring the spectra without capsules. To study the influence of the number density of capsules on the reflectance spectra, we used the same × 50 lens without a field stop. For both cases, spectra from the capsules were normalized with spectra from a broadband mirror (BBDS-PM-1037-0, CVI Laser, LLC). Thickness of solid or rubber capsule membranes and arrangement of colloids in the capsules are characterized by SEM (Ultra55, Zeiss). How to cite this article: Kim, S.-H. et al . Osmotic-pressure-controlled concentration of colloidal particles in thin-shelled capsules. Nat. Commun. 5:3068 doi: 10.1038/ncomms4068 (2014).